Cholesterol modulates cell signaling and protein networking by specifically interacting with PDZ domain-containing scaffold proteins Cholesterol is known to modulate the physical properties of cell membranes, but its direct involvement in cellular signaling has not been thoroughly investigated. Here we show that cholesterol specifically binds many PDZ domains found in scaffold proteins, including the N-terminal PDZ domain of NHERF1/EBP50. This modular domain has a cholesterol-binding site topologically distinct from its canonical protein-binding site and serves as a dual-specificity domain that bridges the membrane and juxta-membrane signaling complexes. Disruption of the cholesterol-binding activity of NHERF1 largely abrogates its dynamic co-localization with and activation of cystic fibrosis transmembrane conductance regulator, one of its binding partners in the plasma membrane of mammalian cells. At least seven more PDZ domains from other scaffold proteins also bind cholesterol and have cholesterol-binding sites, suggesting that cholesterol modulates cell signaling through direct interactions with these scaffold proteins. This mechanism may provide an alternative explanation for the formation of signaling platforms in cholesterol-rich membrane domains. Regulation of cellular processes, such as cell signaling, involves a myriad of protein–protein interactions. Cellular membranes, the plasma membrane (PM) in particular, offer unique local environments for effective protein–protein interactions and therefore serve as the main sites for protein complexes and networks [1] , [2] , [3] . Accumulating evidence suggests that membrane lipids have a critical role in spatiotemporal regulation of protein networking on or near membranes through direct interactions with signaling proteins [3] , [4] . The inner leaflet of PM of mammalian cells contains various lipids, such as phosphatidylserine (PS) [5] , [6] and phosphatidylinositol (PI)-4,5-trisphosphate (PtdIns(4,5)P 2 ) [7] , [8] , that can serve as site-specific membrane signals for recruiting cellular proteins and modulating their individual function and mutual interactions. It can also transiently produce lipids, such as PI-3,4,5-bisphosphate or diacylglycerol, which have key signaling roles. Cholesterol is a major (that is, 30–40%) lipid component of the mammalian PM whose cellular concentration is tightly regulated. Although much is known about the metabolism and transport of cholesterol and its role in atherosclerosis [9] , less is known about the exact cellular functions of cholesterol. Cholesterol has been implicated in the regulation of physical properties of the membrane, most notably the formation of cholesterol-rich lipid rafts [10] , the modulation of the activities of some integral membrane proteins [11] , [12] , [13] and the regulation of cellular proteins through the oxysterol-binding protein [14] ; however, its direct involvement in cellular processes, cell signaling in particular, through specific interactions with the components of the major signaling pathways has not been thoroughly investigated. Here we show that cholesterol binds with high affinity and specificity to Postsynaptic density 95, Disc large 1, and Zonular occludens 1 (PDZ) domains of many scaffold proteins, including NHERF1/EBP50, which have key roles in protein networking, and that these interactions are essential for their cellular and physiological functions. Many PDZ domains bind cholesterol Modular protein-interaction domains (PIDs) have important roles in protein interactions and networking during cell signaling [15] , [16] , [17] . To identify new cholesterol-binding proteins that regulate cell signaling, we therefore set out to screen PIDs for cholesterol-binding activity by surface plasmon resonance (SPR) analysis. The PDZ domain is a small (≈90 amino acids) modular PID that reversibly interacts with a short hydrophobic C-terminal sequence of its target proteins [18] , [19] . PDZ domains have high similarity in terms of both amino-acid sequence and tertiary structure. Among PIDs, we focused on the PDZ domain for three reasons. First, most PDZ domain-containing proteins have multiple copies of PDZ domains and other modular domains, serving as prototype scaffold proteins that dynamically coordinate signaling complex formation and protein networking [18] , [19] . Second, many PDZ domains have been reported to interact with membrane lipids [20] , [21] , [22] , [23] , [24] , [25] . Third, we found that many PDZ domains contain a cholesterol-recognition amino-acid consensus (CRAC) motif ( L/V -(X)(1–5)- Y -(X)(1–5)- R/K -, in which (X)(1–5) represents one to five residues of any amino acid) that has been identified in several cholesterol-binding integral membrane proteins [26] , but not in cytosolic proteins. Sequence analysis of PDZ domains reveals that among 144 mouse PDZ domains, 49 of them (≈34%) contain one or more CRAC motif (see Supplementary Table S1 ), suggesting that they may bind cholesterol. Because cholesterol is mainly found in the PM, we first screened for the PDZ domains with high affinity for the vesicles whose lipid composition recapitulate the cholesterol-rich inner PM of mammalian cells (see Methods) and assessed their cholesterol specificity by determining cholesterol dependency in membrane binding. Screening of 30 available PDZ domains among those listed in Supplementary Table S1 by SPR analysis showed that 12 PDZ domains have submicromolar affinity for the PM-mimetic vesicles, and that 8 of them show definite cholesterol dependency in membrane binding, albeit to varying degrees (see Supplementary Fig. S1 ). They include the PDZ domains from NHERF1/EBP50, 3 syntrophin isoforms (α, β2 and γ2), tamalin, PDZK2, PSD95 and SAP97, all of which are well-characterized scaffold/adaptor proteins. These proteins show significantly reduced binding when cholesterol was either replaced by a cholesterol derivative, 5α,6β-dihydroxycholestanol, or removed from the PM-mimetic vesicles. The list of cholesterol-binding PDZ domains is expected to grow as more PDZ domains in Supplementary Table S1 are tested for cholesterol dependency. Collectively, our results show that a large proportion of PDZ domains from various cellular proteins with diverse functions bind PM with high affinity and in a cholesterol-dependent manner. NHERF1-PDZ1 domain specifically binds cholesterol Among cholesterol-binding PDZ domains, the N-terminal PDZ domain (PDZ1) of NHERF1 showed the highest affinity for the PM-mimetic vesicles (that is, K d ≈40 nM; see Supplementary Fig. 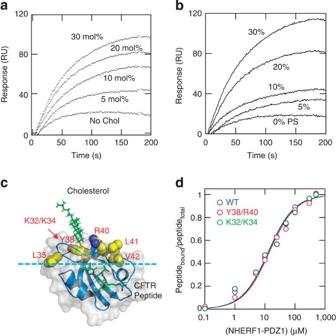Figure 1: Lipid binding of NHERF1-PDZ1 domain. (a) Cholesterol dependence and (b) PS dependence of membrane binding of NHERF1-PDZ1. The PDZ domain (300 nM) was allowed to interact with POPC/cholesterol/POPS (80-x:20:xor 80-x:x:20) vesicles. (c) A model structure of the NHERF1–PDZ1–cholesterol-peptide ternary complex. Docking of a cholesterol molecule and a C-terminal CFTR peptide (QDTLR) to the NHERF1-PDZ1 (PDB ID: 1G9O) was performed as described inSupplementary Information. Cholesterol (with its hydrophobic tail pointing upward) and the bound peptide are shown in stick representation. The side chains of putative cholesterol-binding, CRAC motif residues, L35, Y38 and R40 are shown in space-filling representation and labelled. The location of the putative anionic lipid-binding site composed of K32 and K34 is indicated by a red arrow. The side chain conformation of K32/K34 is not fully resolved in the crystal structure, which hampered the modeling with a bound PS molecule. Also shown are L41 and V42 that may be involved in membrane penetration. The structure is shown in a putative membrane-binding orientation with the dotted line indicating the membrane surface. Notice that the putative lipid binding sites are topologically distinct from the peptide-binding pocket. The model was built in the absence of the lipid bilayer and the membrane-bound protein may undergo further conformational changes. (d) Effects of mutations of NHERF1-PDZ1 on its CFTR peptide binding. Binding of WT (blue), K32A/K34A (green) and Y38A/R40A (red) to F-Ahx-VQDTLR was monitored by fluorescence anisotropy. Notice that mutations have little to no effect on peptide binding (Kd=13±1 μM for WT, 13±2 μM for K32A/K34A and 14±1 μM for Y38A/R40A); see Methods for experimental details. S2 and Table 1 ) and the most pronounced cholesterol dependency in membrane binding ( Fig. 1a ). We therefore performed detailed functional studies on the NHERF1-PDZ1 domain and the full-length NHERF1. NHERF1-PDZ1 bound radiolabelled cholesterol with 1:1 stoichiometry ( Supplementary Fig. S3 ) and showed much lower binding to other related lipids, such as two oxysterols or ceramide, demonstrating its cholesterol specificity ( Supplementary Fig. S4 ). Cholesterol-dependent membrane binding of NHERF1-PDZ1 was further supported by direct quantitative fluorescence imaging of enhanced green fluorescence protein (EGFP)-tagged NHERF1-PDZ1 bound to giant unilamellar vesicles (GUVs) containing various concentrations of cholesterol (see Supplementary Fig. S5 ). The full-length NHERF1 also bound cholesterol-containing membranes with high affinity and specificity, and truncation of the PDZ1 domain from NHERF1 abrogated the cholesterol-dependent membrane binding ( Table 1 ). NHERF1 has another PDZ domain (PDZ2) in the C-terminal end of the PDZ1 domain but it shows no membrane affinity ( Table 1 ). Table 1 Membrane-binding properties of NHERF1, their PDZ domains and mutants measured by SPR analysis. Full size table Figure 1: Lipid binding of NHERF1-PDZ1 domain. ( a ) Cholesterol dependence and ( b ) PS dependence of membrane binding of NHERF1-PDZ1. The PDZ domain (300 nM) was allowed to interact with POPC/cholesterol/POPS (80- x :20: x or 80- x : x :20) vesicles. ( c ) A model structure of the NHERF1–PDZ1–cholesterol-peptide ternary complex. Docking of a cholesterol molecule and a C-terminal CFTR peptide (QDTLR) to the NHERF1-PDZ1 (PDB ID: 1G9O) was performed as described in Supplementary Information . Cholesterol (with its hydrophobic tail pointing upward) and the bound peptide are shown in stick representation. The side chains of putative cholesterol-binding, CRAC motif residues, L35, Y38 and R40 are shown in space-filling representation and labelled. The location of the putative anionic lipid-binding site composed of K32 and K34 is indicated by a red arrow. The side chain conformation of K32/K34 is not fully resolved in the crystal structure, which hampered the modeling with a bound PS molecule. Also shown are L41 and V42 that may be involved in membrane penetration. The structure is shown in a putative membrane-binding orientation with the dotted line indicating the membrane surface. Notice that the putative lipid binding sites are topologically distinct from the peptide-binding pocket. The model was built in the absence of the lipid bilayer and the membrane-bound protein may undergo further conformational changes. ( d ) Effects of mutations of NHERF1-PDZ1 on its CFTR peptide binding. Binding of WT (blue), K32A/K34A (green) and Y38A/R40A (red) to F-Ahx-VQDTLR was monitored by fluorescence anisotropy. Notice that mutations have little to no effect on peptide binding ( K d =13±1 μM for WT, 13±2 μM for K32A/K34A and 14±1 μM for Y38A/R40A); see Methods for experimental details. Full size image Because little is known about the mechanism by which cytosolic proteins interact with cholesterol, we performed detailed biophysical studies to elucidate the mechanism of cholesterol binding by NHERF1-PDZ1. Cholesterol is a largely hydrophobic molecule with a small polar headgroup, it is thus located close to the hydrophobic core of the lipid bilayer and should not be readily accessible from outside. For this reason, binding of PDZ domains to cholesterol in the PM should involve partial membrane penetration of hydrophobic protein residues into the interior of the membrane [27] , which typically follows initial membrane association driven by electrostatic interactions between cationic protein residues and anionic lipids [28] , such as PS. Binding of PDZ domains to anionic lipids has been well documented [20] , [23] , [25] . To see if the NHERF1-PDZ1 domain follows this mechanism, we first measured its anionic lipid dependence. As illustrated in Fig. 1b , NHERF1-PDZ1 interacts with anionic phospholipids, including PS, in a concentration-dependent manner, and this interaction is non-specific in nature because NHERF1-PDZ1 can also interact with other anionic lipids equally well (see Supplementary Fig. S4 ). In the absence of PS (or other anionic lipids) in the vesicles, NHERF1-PDZ1 had much reduced binding to cholesterol-containing vesicles, showing that this non-specific electrostatic interaction is required for ensuing cholesterol binding. We also found that NHERF1-PDZ1 was capable of penetrating the cholesterol-containing lipid monolayer, which was again facilitated by PS binding (see Supplementary Fig. S6 ). Collectively, these results show that NHERF1-PDZ1 specifically binds cholesterol and that non-specific anionic lipid binding and subsequent membrane penetration are essential for its cholesterol binding. NHERF1-PDZ1 has separate lipid and protein-binding sites We then mapped the anionic lipid and cholesterol-binding sites of the PDZ domain by molecular modeling and mutational analysis. NHERF1-PDZ1 contains a CRAC motif in residues 35–40 (LGQYIR). Mutation of L35, Y38 and R40 reduced the membrane affinity of the NHERF1-PDZ1, albeit to varying degrees ( Table 1 ). A double-site mutant Y38A/R40A had 18-fold lower affinity than wild type (WT) NHERF1-PDZ1 for the PM-mimetic vesicles ( Table 1 ). It also showed dramatically reduced binding to radiolabelled cholesterol ( Supplementary Fig. S3A ), and no cholesterol dependency in membrane binding ( Supplementary Fig. S3B ), indicating that Y38 and R40 are involved in specific cholesterol binding and that this mutant can be used as a cholesterol-binding-deficient variant in further studies. The mutation Y38A/R40A exerted the same negative effect on membrane binding of the full-length NHERF1 ( Table 1 ). The molecular surface surrounding the CRAC motif contains cationic (for example, K32 and K34) and hydrophobic (for example, L41 and V42) residues ( Fig. 1c ), suggesting that they might be involved in anionic lipid binding and partial membrane penetration, respectively. Mutational analysis confirmed that all these residues significantly contribute to membrane binding of NHERF1-PDZ1 ( Table 1 ). Specifically, K32A/K43A showed greatly reduced binding to PS-containing membranes and much reduced PS dependency compared with the WT ( Supplementary Fig. S7 ). This indicates that K32 and K34 are involved in anionic lipid binding. Also, L41 and V42 appear to be involved in membrane penetration of NHERF1-PDZ1 as L41A and V42A exhibited lower-membrane penetration activity than the WT when measured by the monolayer penetration assay ( Supplementary Fig. S6 ). Molecular modeling (see Supplementary Methods ) based on these mutational data suggests that the putative lipid-binding sites of NHERF1-PDZ1 are completely separate from its canonical protein-binding pocket and that NHERF1-PDZ1 can bind lipids and the peptide simultaneously ( Fig. 1c ). This notion was verified by the finding that neither Y38A/R40A nor K32A/K34A mutation had significant effect on the interaction of NHERF1-PDZ1 with the C-terminal peptide (that is, VQDTLR) of its binding partner, cystic fibrosis transmembrane conductance regulator (CFTR) [29] , in a fluorescence anisotropy assay ( Fig. 1d ). The mutations also had negligible effects on the peptide binding of the full-length NHERF1 when measured by a glutathione- S -transferase pull-down assay ( Supplementary Fig. S8 ). The independence of lipid- and protein-binding sites of NHERF1-PDZ1 is further supported by the findings that the CFTR peptide showed a negligible effect on the binding of NHERF1-PDZ1 to PM-mimetic vesicles ( Supplementary Fig. S9A ) and that the presence of PM-mimetic vesicles did not significantly interfere with the binding of NHERF1-PDZ1 to the CFTR peptide ( Supplementary Fig. S9B ). CFTR contains negatively charged residues immediately preceding the PDZ-binding motif ( EE T EEE VQDTRL) that may interfere with interaction between NHERF1-PDZ1 and anionic lipids in the membrane when the intact CFTR molecule forms a complex with NHERF1. To investigate this potential inhibitory effect of the anionic patch, we first built a structural model of the C-terminal domain of CFTR (residues 1423–1480; referred to as CFTR-14) that includes the anionic patch and the PDZ domain-binding motif complexed with NHERF1-PDZ1 (see Supplementary Fig. S10A ) and calculated the electrostatic potential of the complex (see Supplementary Fig. S10B ). The calculation suggests that despite the presence of the anionic patch, the overall electrostatic profile of the complex remains largely positive, particularly on the putative membrane-binding surface, because the negative contribution of the anionic patch is canceled out by the cationic residues on the helix at the end of CFTR-14. We also performed the binding measurements with an extended C-terminal peptide (EETEEEVQDTRL). The extended peptide had essentially the same affinity as the shorter one (that is, VQDTLR) for NHERF1-PDZ1 ( Supplementary Fig. S11A ) and did not inhibit the binding of NHERF1-PDZ1 to PM-mimetic vesicles ( Supplementary Fig. S11C ). Also, the presence of PM vesicles did not interfere with binding of the extended peptide to NHERF1-PDZ1 ( Supplementary Fig. S11B ). Collectively, these findings suggest that the anionic patch in CFTR would not interfere with the NHERF1-PDZ1-membrane interaction proposed in Fig. 1c . Cholesterol binding is mediated through the CRAC motif To test if the CRAC motif is also responsible for cholesterol binding of other PDZ domains, we further characterized α-syntrophin-PDZ. As shown in Fig. 2a , membrane binding of α-syntrophin-PDZ depended on the concentration of cholesterol in the membrane. α-syntrophin-PDZ has a CRAC motif ( L EVK Y M K ) and the relative side chain orientation of Y162 and K164 of α-syntrophin is similar to that of Y38 and R40 of NHERF1-PDZ1 [30] . Indeed, when Y162 and K164 of α-syntrophin-PDZ were mutated to Ala, the Y162A/K164A mutant showed little cholesterol dependency in membrane binding ( Fig. 2b ) and, consequently, had much lower affinity than the WT at higher cholesterol concentrations. The mutant and the WT had comparable affinity for non-cholesterol-containing vesicles, indicating that the mutant is structurally intact and has basal membrane-binding activity. This suggests that the CRAC motif in general is involved in the cholesterol binding of PDZ domains. 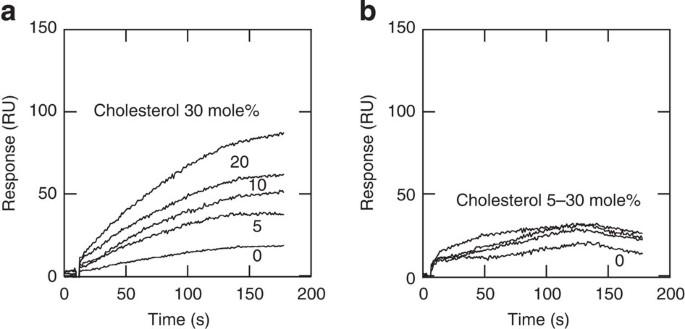Figure 2: Membrane binding of α-syntrophin PDZ domain and its CRAC motif mutant. (a) Cholesterol dependence of membrane binding of α-syntrophin-PDZ. (b) Cholesterol dependence of membrane binding of α-syntrophin-PDZ Y162A/K164A. The conditions are the same as described forFig. 1a: that is, the PDZ domain (300 nM) was allowed to interact with POPC/cholesterol/POPS (80-x:x:20) vesicles. Notice that the mutant shows much lower resonance units (RUs), little cholesterol dependency and altered binding curves, all consistent with its reduced cholesterol binding. Figure 2: Membrane binding of α-syntrophin PDZ domain and its CRAC motif mutant. ( a ) Cholesterol dependence of membrane binding of α-syntrophin-PDZ. ( b ) Cholesterol dependence of membrane binding of α-syntrophin-PDZ Y162A/K164A. The conditions are the same as described for Fig. 1a : that is, the PDZ domain (300 nM) was allowed to interact with POPC/cholesterol/POPS (80- x : x :20) vesicles. Notice that the mutant shows much lower resonance units (RUs), little cholesterol dependency and altered binding curves, all consistent with its reduced cholesterol binding. Full size image NHERF1-cholesterol binding is essential for its activity To establish the physiological significance of cholesterol–NHERF1 binding, we measured the effect of suppressing cholesterol binding of NHERF1 on its cellular functions. NHERF1 is a multi-domain scaffold protein that interacts with diverse integral membrane proteins, including CFTR and β2-adrenergic receptor, and cytosolic proteins [31] , [32] . Because NHERF1 is known to mediate the activation of CFTR by protein kinase A (PKA) by serving as a scaffold for these proteins [29] , we measured the chloride channel activity of CFTR as an indirect cellular activity assay for NHERF1. We first measured the effect of exogenous expression of NHERF1 WT and Y38A/R40A on the activity of CFTR in HEK293 cells expressing CFTR using the whole-cell patch clamp ( Fig. 3a ). Expression of NHERF1 WT did not evoke a significant increase in forskolin-induced Cl − current over control cells, presumably, due to the presence of the endogenous NHERF1 in HEK293 cells. Interestingly, expression of the Y38A/R40A mutant, which has compromised cholesterol-binding activity while having intact CFTR-binding activity, decreased CFTR-mediated Cl − current by 48.5%, indicating that the mutant exerts a dominant-negative effect because of its inability to bind cholesterol effectively. Furthermore, reduction of the cholesterol level of HEK293 cells by cholesterol oxidase treatment significantly lower the CFTR activity in NHERF1 WT-expressing cells, but not in Y38A/R40A-expressing cells, confirming the importance of cholesterol in NHERF1-mediated CFTR activation. 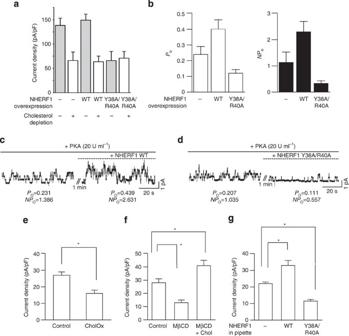Figure 3: Effects of cholesterol on the cellular activities of NHERF1. (a) Whole-cell CFTR current was measured in CFTR-overexpressing HEK293 cells that were co-transfected with various NHERF1 constructs. Peak currents were normalized as currents densities (pA/pF), and each bar represents the average and the s.e. from >9 experiments. The cholesterol depletion was performed by treating a batch of in HEK293 cells with cholesterol oxidase (1 U ml−1) for 1 h at 37 °C. (b) Single CFTR channel activity in the presence of NHERF1 WT and Y38A/R40A. CFTR Cl−channel activity was measured in CFTR-transfected HEK293 cells with inside-out configurations. Each bar represents the average and the s.e. from >6 experiments. (c,d) Representative traces of CFTR single-channel measurements showing the effect of NHERF1 WT and Y38A/R40A on CFTR channel activity, respectively. Current records at −60 mV were analysed to estimate thePo. After a 5-min wash of patch membranes, CFTR was activated by addition of PKA and ATP (3 mM). Solutions containing purified NHERF1 proteins (100 nM) were perfused to the bath chamber for 5 min.PoandNPowere calculated from the recording of the last 3 min of each 5-min interval. (e,f) Whole-cell CFTR currents were measured in colonic T84 cells, which natively express CFTR and NHERF1. Each bar represents the average and the s.e. from >10 experiments. Cells were treated with cholesterol oxidase (1 U ml−1), MβCD (100 μM) or cholesterol-loaded MβCD (100 μM) for 1 h at 37 °C. Asterisks indicateP<0.01. (g) CFTR channel activity was measured with patch pipettes containing recombinant NHERF1 WT and Y38A/R40A proteins (100 nM). Currents were measured after a 10-min equilibration with pipette solution that contained each recombinant protein. Each bar represents the average and the s.e. from six experiments. Asterisks indicateP<0.05. Figure 3: Effects of cholesterol on the cellular activities of NHERF1. ( a ) Whole-cell CFTR current was measured in CFTR-overexpressing HEK293 cells that were co-transfected with various NHERF1 constructs. Peak currents were normalized as currents densities (pA/pF), and each bar represents the average and the s.e. from >9 experiments. The cholesterol depletion was performed by treating a batch of in HEK293 cells with cholesterol oxidase (1 U ml −1 ) for 1 h at 37 °C. ( b ) Single CFTR channel activity in the presence of NHERF1 WT and Y38A/R40A. CFTR Cl − channel activity was measured in CFTR-transfected HEK293 cells with inside-out configurations. Each bar represents the average and the s.e. from >6 experiments. ( c , d ) Representative traces of CFTR single-channel measurements showing the effect of NHERF1 WT and Y38A/R40A on CFTR channel activity, respectively. Current records at −60 mV were analysed to estimate the P o . After a 5-min wash of patch membranes, CFTR was activated by addition of PKA and ATP (3 mM). Solutions containing purified NHERF1 proteins (100 nM) were perfused to the bath chamber for 5 min. P o and NP o were calculated from the recording of the last 3 min of each 5-min interval. ( e , f ) Whole-cell CFTR currents were measured in colonic T84 cells, which natively express CFTR and NHERF1. Each bar represents the average and the s.e. from >10 experiments. Cells were treated with cholesterol oxidase (1 U ml −1 ), MβCD (100 μM) or cholesterol-loaded MβCD (100 μM) for 1 h at 37 °C. Asterisks indicate P <0.01. ( g ) CFTR channel activity was measured with patch pipettes containing recombinant NHERF1 WT and Y38A/R40A proteins (100 nM). Currents were measured after a 10-min equilibration with pipette solution that contained each recombinant protein. Each bar represents the average and the s.e. from six experiments. Asterisks indicate P <0.05. Full size image To minimize the effects of the endogenous NHERF1 in HEK293 cells, we also measured the single CFTR channel activity using inside-out configurations. When CFTR was treated with catalytic subunit of PKA and ATP to the bath solution, an ion channel activity with a single-channel conductance of 7.1±0.3 pS and a linear current-voltage relationship was evoked that was absent in mock-transfected cells ( Fig. 3c ). Treatment with the purified NHERF1 WT protein (100 nM) to the bath (cytosolic side in inside-out configuration) induced 1.7-fold and 2.0-fold increases in the open probability ( P o ) and NP o of CFTR, respectively ( Fig. 3b ). In contrast, the addition of the Y38A/R40A mutant protein (100 nM) decreased the P o and NP o of CFTR by 50.7% and 34.6% ( Fig. 3b ), respectively, showing that the cholesterol-binding-deficient NHERF1 mutant has an intrinsic CFTR-inhibitory activity, which is consistent with its dominant-negative effect seen in the whole patch experiment. To further demonstrate the physiological relevance of the cholesterol–NHERF1 binding, we measured the CFTR channel activity of colonic T84 cells that endogenously express CFTR and NHERF1. It was previously reported that genetic ablation of NHERF1 reduced CFTR-mediated anion secretion by 47.6% in mouse intestines, showing the importance of NHERF1 in CFTR activation under physiological conditions [33] . When we treated T84 cells with cholesterol oxidase or methyl-β-cyclodextrin (MβCD) to suppress the cholesterol level, the CFTR channel activity in T84 cells was decreased by 40–50% ( Fig. 3e ). Supplementation of cholesterol to the cells by treatment with cholesterol-loaded MβCD restored the channel activity, indicating that the current reduction by MβCD was not due to the nonspecific toxic effect of MβCD ( Fig. 3e ). Comparable levels of reduced CFTR channel activity by NHERF1 gene knockout and cholesterol depletion suggest that cholesterol binding is essential for the activation of CFTR by NHERF1. Furthermore, when we performed whole-cell current recordings in T84 cells with a pipette containing recombinant NHERF1 proteins, inclusion of NHERF1 WT in the pipette solution resulted in a 1.5-fold increase in CFTR currents within 10 min of membrane rupture by patch pipette ( Fig. 3g ). However, inclusion of NHERF1 Y38A/R40A in the patch pipette attenuated the activity of native CFTR in T84 cells by 50.5% ( Fig. 3g ), again confirming the dominant-negative effect of this mutant protein. Presumably, treatment of T84 cells with NHERF1 Y38A/R40A reduces CFTR currents by interfering with the cholesterol-dependent interaction between endogenous NHERF1 and CFTR. Taken together, these results underscore the critical role of cholesterol binding in the NHERF1-mediated regulation of CFTR activity. Cholesterol regulates co-localization of signaling proteins In general, lipids serve as membrane-specific signals that drive or promote the membrane recruitment of their effector proteins containing lipid-binding domains or motifs [27] , [34] , [35] . Confocal imaging showed that the mutation of anionic lipid-binding residues (K32A/K34A) abrogated the PM localization of the EGFP-tagged full-length NHERF1 ( Fig. 4a ), although the mutation did not alter its affinity for its protein partner, CFTR, at the PM ( Fig. 1d ). It is thus clear that anionic lipid binding is important for its PM localization. Interestingly, the mutations of cholesterol-binding residues in NHERF1 (Y38A/R40A) did not significantly change its PM localization patterns ( Fig. 4a ), suggesting that cholesterol binding does not drive the PM localization per se but may have a more subtle regulatory role. 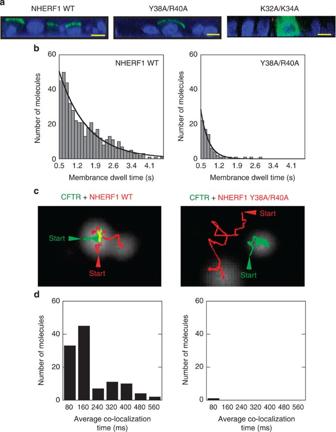Figure 4: Regulation of signaling protein localization by cholesterol. (a) Confocal images of EGFP-NHERF1 full-length WT, K32A/K34A and Y38A/R40A transiently expressed in MDCK2 cells. Three days after plating onto Transwell filter, cells were subjected to immunofluorescence analysis. NHERF1 was visualized by EGFP (green) and the nucleus by DAPI staining (blue). Notice that WT and Y38A/R40A are localized at the apical PM, whereas K32A/K34A show diffuse cytosolic distribution. About 80% of 40–50 cells examined for each protein showed the same patterns as these representative images. Scale bars indicate 10 μm. (b) Distribution of membrane dwell time of Halo-TMR-NHERF1 full-length WT and Y38A/R40A determined by TIRF single-molecule imaging. The number of NHERF1 molecules (N) spending a given time (t) on the PM of HEK293 cells stably expressing EGFP-CFTR is displayed. The solid curves are best fits to the single exponential decay equation:N=Nox e−ktwherekindicates the membrane dissociation rate constant.k=1.0±0. 1 s−1for WT and 3.7±0.2 s−1for Y38A/R40A. Notice that WT has a much larger membrane population and a longer membrane residence time (that is, smallerk) than Y38A/R40A. (c) A representative pair of NHERF1 and CFTR is shown for NHERF1 WT and Y38A/R40A, respectively. Many NHERF1 WT molecules show dynamic co-localization with CFTR, whereas most of Y38A/R40A molecules exhibit separate localization with CFTR. White dots indicate individual molecules and red and green lines are trajectories for NHERF1 and CFTR, respectively. (d) Distribution of co-localization time of CFTR with NHERF1 WT and Y38A/R40A determined under the same conditions. The number of CFTR molecules spending a given co-localzation time with NHERF1 WT (within 100 nm distance) on the PM of HEK293 cells is displayed. Notice that a significant portion of CFTR molecules are co-localized with NHERF1 WT for >300 ms. In contrast, no CFTR molecule was found to co-localized with the NHERF1 Y38A/R40A mutant for >100 ms. Figure 4: Regulation of signaling protein localization by cholesterol. ( a ) Confocal images of EGFP-NHERF1 full-length WT, K32A/K34A and Y38A/R40A transiently expressed in MDCK2 cells. Three days after plating onto Transwell filter, cells were subjected to immunofluorescence analysis. NHERF1 was visualized by EGFP (green) and the nucleus by DAPI staining (blue). Notice that WT and Y38A/R40A are localized at the apical PM, whereas K32A/K34A show diffuse cytosolic distribution. About 80% of 40–50 cells examined for each protein showed the same patterns as these representative images. Scale bars indicate 10 μm. ( b ) Distribution of membrane dwell time of Halo-TMR-NHERF1 full-length WT and Y38A/R40A determined by TIRF single-molecule imaging. The number of NHERF1 molecules ( N ) spending a given time ( t ) on the PM of HEK293 cells stably expressing EGFP-CFTR is displayed. The solid curves are best fits to the single exponential decay equation: N = N o x e −kt where k indicates the membrane dissociation rate constant. k =1.0±0. 1 s −1 for WT and 3.7±0.2 s −1 for Y38A/R40A. Notice that WT has a much larger membrane population and a longer membrane residence time (that is, smaller k ) than Y38A/R40A. ( c ) A representative pair of NHERF1 and CFTR is shown for NHERF1 WT and Y38A/R40A, respectively. Many NHERF1 WT molecules show dynamic co-localization with CFTR, whereas most of Y38A/R40A molecules exhibit separate localization with CFTR. White dots indicate individual molecules and red and green lines are trajectories for NHERF1 and CFTR, respectively. ( d ) Distribution of co-localization time of CFTR with NHERF1 WT and Y38A/R40A determined under the same conditions. The number of CFTR molecules spending a given co-localzation time with NHERF1 WT (within 100 nm distance) on the PM of HEK293 cells is displayed. Notice that a significant portion of CFTR molecules are co-localized with NHERF1 WT for >300 ms. In contrast, no CFTR molecule was found to co-localized with the NHERF1 Y38A/R40A mutant for >100 ms. Full size image To better understand the role of cholesterol binding in the function of NHERF1, we performed dual-colour single-molecule tracking of NHERF1 and CFTR by total internal reflection fluorescence (TIRF) microscopy. It has been well documented that single-molecule tracking can sensitively and accurately detect dynamic, transient interactions among a small population of proteins that typically occur during cell signaling but cannot be detected by conventional bulk imaging methods, such as confocal imaging [36] . For these studies, NHERF1 was fused with the Halo-tag, which can be specifically labelled with tetramethylrhodamine (TMR) in situ and is preferred over red fluorescence proteins for cellular single-molecule measurements [37] , transfected into HEK293 cells stably expressing EGFP-tagged CFTR and labelled with Halo-TMR. First, single-molecule tracking of NHERF1 WT and Y38A/R40A showed that under the same conditions, the WT has a higher membrane population and a longer membrane-residence time than Y38A/R40A ( Fig. 4b ). This is consistent with 20-fold higher membrane affinity of the WT (see Table 1 ) and its ability to partially penetrate the cholesterol-containing membranes ( Supplementary Fig. S6 ). Despite the essentially same chemical affinity of the PDZ1 domains of WT and Y38A/R40A for CFTR (see Fig. 1d ), this favourable membrane-binding activity should allow WT a much better chance to interact and comigrate with CFTR that is present in the PM. Dual-colour single-molecule tracking confirms this notion. That is, a large portion of NHERF1 WT (red) and CFTR (green) molecules co-localize and co-migrate in the PM for a significant period of time ( Fig. 4c ; see also Supplementary Movie S1 ). Under the same conditions, however, the population of NHERF1 Y38A/R40A comigrating with CFTR was much smaller ( Fig. 4c ; see also Supplementary Movie S2 ). The same pattern was seen in >50 different cells. These results indicate that cholesterol-binding activity of NHERF1-PDZ1 is essential for dynamic and sustained co-localization of NHERF1 and CFTR, which should be critical for its regulation of CFTR activity. Our results clearly show that a scaffold protein, NHERF1, specifically interacts with cholesterol in the PM via its PDZ1 domain. The cholesterol-binding site of NHERF1-PDZ1 belongs to the CRAC motif that has been found in many cholesterol-interacting membrane proteins [26] , but not in cytosolic signaling proteins. The cholesterol-binding site of NHERF1-PDZ1 is surrounded by hydrophobic and cationic residues. The cationic residues are necessary for the NHERF1-PDZ1 to interact with anionic lipids, including PS, which drives its initial membrane binding. Upon initial membrane binding, the hydrophobic residues partially penetrate the hydrophobic interior of the membrane, as evidenced by our monolayer penetration data, and this step is necessary for cholesterol binding because cholesterol is buried in the hydrophobic core of the membrane. This complex mechanism of cholesterol binding indicates that for cytosolic proteins, the CRAC motif alone is not sufficient for effective cholesterol binding; proper arrangement of cationic and hydrophobic residues surrounding their cholesterol-binding sites is also necessary. This is because none of the CRAC motifs found in cytosolic proteins, including all PDZ domains, form a conventional, well-defined lipid-binding pocket as seen with other lipid-binding domains, such as PH domain. Thus, proper alignment of hydrophobic and polar residues near the CRAC motif may be critically important for specific binding of cholesterol through hydrogen bonds and hydrophobic contact. In fact, NHERF1-PDZ2 shows little affinity for the PM-mimetic vesicles, despite having a highly similar sequence in the CRAC motif (GQFIR instead of GQYIR of NHERF1-PDZ1), because it lacks hydrophobic residues surrounding the region. Even when Phe in PDZ2 is mutated to Tyr (that is, F178Y-PDZ2), the mutant still shows negligible affinity for PM-mimetic vesicles. For NHERF1-PDZ1, these adjacent cholesterol- and other lipid-binding sites are separate from the canonical peptide-binding pocket, and our experimental and computational results support that NHERF1-PDZ1 can bind the protein and lipids simultaneously. Our partial screening of available PDZ domains revealed that many other CRAC motif-containing PDZ domains, all of which are established scaffold/adaptor proteins, bind the membrane in a cholesterol-dependent manner. These PDZ domains also have cationic and hydrophobic residues surrounding their CRAC motifs. As is the case with NHERF1-PDZ1 and α-syntrophin-PDZ, their CRAC motif is thus likely to be involved in their cholesterol specificity. The molecular location of the CRAC motif within these PDZ domains varies significantly with respect to the canonical peptide-binding pocket, suggesting that cholesterol binding may have different effects on the protein binding and the cellular function of PDZ domains and their host proteins. Collectively, our results provide the first experimental evidence that cholesterol can directly and specifically interact with diverse cytosolic proteins in addition to specialized cholesterol-transfer proteins. Although more studies are needed to gain further mechanistic insight into the order and the interplay of cholesterol and protein binding, our results suggest that these scaffold proteins serve as cholesterol-specific, lipid- and protein-binding modules that can bridge the membrane and diverse juxta-membrane signaling complexes and networks. Our in-depth functional studies of NHERF1 illustrate how cholesterol binding by its PDZ1 domain modulates the cellular signaling activity of this protein. It has been well documented that anionic lipids in the PM of mammalian cells, PS [5] , [6] and PtdIns(4,5)P 2 (refs 7 , 8 ) in particular, have a key role in the PM localization of various cytosolic proteins, including small G proteins. Our results also show that anionic lipid binding is important for the PM localization of NHERF1-PDZ1. Unlike these anionic lipids, cholesterol does not seem to drive the PM localization per se of NHERF1, as expected from the internal location of cholesterol in the membrane, but instead modulates its dynamic and functional co-localization with an interacting partner at the PM. Dual-colour single-molecule tracking of NHERF1 and CFTR shows that cholesterol is essential for sustained dynamic co-localization of these interacting protein partners. In general, modular PIDs, such as the PDZ domain, mediate reversible, low-affinity (that is, high micromolar) and transient interactions among signaling proteins [3] , [15] , [16] , [17] . Because cholesterol binding of a protein entails its membrane penetration ( Supplementary Fig. S6 ), which in general allows its elongated membrane residence (see Fig. 4b ) [27] , cholesterol binding of PDZ domains should naturally facilitate sustained co-localization with their interaction partners at the PM. A recent study showed that cellular signal transduction requires sustained co-localization and transient immobilization of interacting proteins [38] . Cholesterol-induced sustained co-localization of scaffold proteins with their interacting proteins at the PM should thus have important functional consequences. The complex mechanism regulating the NHERF1–CFTR interaction through phosphorylation and protein oligomerization is not fully understood [39] , [40] . Regardless of the mechanism, it is likely that cholesterol binding of NHERF1-PDZ1 reinforces the relatively weak and transient interaction between NHERF1 and CFTR and also helps bring another key signaling molecule, PKA, in the proximity through scaffolding effect, resulting in activation of CFTR. Our cell studies under various conditions confirm the physiological relevance and significance of specific cholesterol binding of NHERF1. Collectively, our study establishes that cholesterol serves as a genuine modulator of cell signaling through its specific interaction with PDZ domain-containing scaffold proteins, including NHERF1. A significant portion of PDZ domains have one or more CRAC motif, and many of them show cholesterol-dependent membrane binding and our bioinformatics search also suggests the presence of the CRAC motif in other PIDs. Thus, cholesterol-dependent cellular regulation via scaffold proteins may represent a new universal mechanism for diverse cell regulation. It has been postulated that cholesterol-rich membrane domains, such as lipid rafts, serve as intracellular signaling and trafficking platforms that recruit multiple membrane and cytosolic proteins [10] . Because cholesterol-binding scaffold proteins organize and coordinate cell-signaling complexes and networks at the PM, our mechanism may provide a complementary or alternative explanation for the cholesterol-mediated formation and regulation of signaling platforms and complexes. As such, our new finding provides an important new clue to understanding complex regulatory mechanisms of cellular signaling and other processes at the PM. Protein preparation All protein constructs containing a C-terminal His 6 tag were bacterially expressed and purified by affinity and ion-exchange chromatography. Protein concentration was then determined by the bicinchoninic acid method (Pierce). Lipid vesicle preparation All lipids were purchased from Avanti Polar Lipids except for the 1,2-dipalmitoyl derivative of PtdIns(4,5)P2 that was from Cayman Chemical. PM-mimetic vesicles were prepared by mixing 1-palmitoyl-2-oleoyl- sn -glycero-3-phosphocholine (POPC), 1-palmitoyl-2-oleoyl- sn -glycero-3-phosphoethanolamine (POPE), 1-palmitoyl-2-oleoyl- sn -glycero-3-phosphoserine (POPS), cholesterol, bovine liver PI and PtdIns(4,5)P 2 in a molar ratio of 12:35:22:22:8:1. The lipid composition of PM-cholesterol vesicles was POPC/POPE/POPS/PI/PtdIns(4,5)P 2 (23:46:22:8:1). Large unilamellar vesicles with 100-nm diameter were prepared with a Liposofast microextruder (Avestin) using a 100-nm polycarbonate filter. Lipid composition of vesicles before and after the extrusion was determined by mass spectrometry (see Supplementary Fig. S13 ) and the cholesterol concentration was slightly (≈18%) reduced after the extrusion. Thus, the effective cholesterol concentration of the extruded PM vesicles was ≈18 mole%. Similar results were obtained for extruded vesicle containing 5α,6β-dihydroxycholestanol (see Fig. S14 ). GUVs were prepared by electroformation as described previously [41] . SPR measurements All SPR measurements were performed at 23 °C in 20 mM Tris–HCl, pH 7.4, containing 0.16 M KCl using a lipid-coated L1 chip in the Biacore X system as described previously [42] , [43] . PM-mimetic (or other) vesicles and POPC vesicles were used as the active and the control surface, respectively. Vesicles were injected at 5 μl min −1 onto the corresponding sensor chip surfaces to yield the identical resonance units, ensuring the equal concentration of the coated lipids. Equilibrium measurements were performed at a flow rate of 5 μl min −1 , which allowed enough time for the R -values of the association phase to reach near equilibrium levels ( R eq ) [44] . Each sensorgram was background-corrected by subtracting the control surface response from the active surface response. A minimum of five different protein concentrations were injected to collect a set of R eq values that were plotted against the protein concentrations ( P o ). An apparent dissociation constant ( K d ) was then determined by nonlinear least-squares analysis of the binding isotherm using the following equation: R eq = R max /(1+ K d / P o ) where R max indicates the maximal R eq value [45] . Because the concentration of lipids coated on the sensor chip cannot be accurately determined, K d is defined as P o yielding half-maximal binding with a fixed lipid concentration. The measurement was repeated at least three times to determine average and s.d. values. For kinetic measurements, the flow rate was maintained from 20 to 30 μl min −1 . Binding to cholesterol-containing GUV Quantitative fluorescence imaging measurements were carried out at 37 °C using a custom-built two-photon microscope as described previously [46] . Binding to radiolabelled cholesterol Binding of PDZ domains to 1,2-3H-labelled cholesterol (Perkin-Elmer) was performed in 20 mM Tris–HCl, pH 7.4, with 160 mM NaCl and 1 μM of protein as reported previously [47] . PDZ–peptide binding assay by fluorescence anisotropy A fluorescein-6-aminohexanoyl (F-Ahx)-labelled peptide, F-Ahx-VQDTLR or F-Ahx-EETEEEVQDTLR, was dissolved in 20 mM Tris buffer, pH 7.9, containing 160 mM NaCl, 300 mM imidazole and 5% dimethylsulfoxide. To each well of Corning 96 flat bottom black polystyrol plate was added 100 μl solution containing each peptide (5 nM final concentration) and each PDZ domain solution (concentration ranging from 100 nM to 1 mM). After incubation for 30 min, the plate was inserted into Tecan Genios Pro spectrofluorometer, and the fluorescence anisotropy ( r ) was measured with excitation and emission wavelengths set at 485 and 535 nm, respectively. Because P o >> Pep o under our conditions, the K d for the PDZ domain–peptide binding was determined by the nonlinear least-squares analysis of the binding isotherm using the equation: where Pep bound , Pep o and P o indicate the concentration of bound peptide, total peptide and total PDZ domain, respectively, and Δr and Δr max are the anisotropy change for each P o and the maximal Δr , respectively. Measurement of chloride channel activity of CFTR Whole-cell and single-channel recordings were performed at room temperature in T84 cells and HEK293 cells expressing CFTR and/or various NHERF1 constructs using the protocols reported previously [48] . After establishing the whole-cell configuration, CFTR was activated by adding forskolin (5 μM). The current output was filtered at 5 kHz and currents were digitized and analysed using AxoScope 10.2 system and Digidata 1322A analog/digital converter (Axon Instruments). The authenticity of currents generated by CFTR was confirmed by control measurements ( Fig. S12 ). Single-channel activity was measured in inside-out configurations using fire-polished pipettes with a resistance of 20–25 megohms. Following patch excision, channels were activated by adding the catalytic subunit of PKA (20 U ml −1 ; Promega) and 3 mM MgATP. After channel activation, purified NHERF1-WT or NHERF1-Y38A/R40A protein (100 nM) was added to the bath. The voltage and current data were low pass-filtered at 0.5 kHz during the recordings, and the single-channel data were further digitally filtered at 25 Hz. It has been shown in excised patches that NHERF1 can directly upregulate CFTR Cl − channel function independently of its AKAP-recruiting scaffold activity [48] . Confocal and single-molecule imaging MDCK2 cells transiently transfected with EGFP-tagged NHERF1 were used for confocal imaging. HEK293 cells stably expressing the EGFP-CFTR with transfected with Halo (Promega)-tagged NHERF-1 and labelled with Halo-Tag TMR (Promega) for TIRF imaging. An Olympus IX71 microscope was used as the base for the custom-built TIRF microscope. The fluorescence from the sample was split into two channels through a dichroic mirror, passed through emission filters and finally projected on to the EM-CCD cameras (Andor) acquiring images of 512 × 512 at 30 ms interval. The images were spatially corrected following the algorithm described previously [36] . All particle tracking, data analysis and image processing were carried out with in-house programs written in MATLAB. The histograms of the length of all the tracks were generated using appropriate bin sizes. Models of PDZ domains in complex with lipids and peptides We first built a model of the PDZ–peptide complex using the crystal structures of the NHERF1-PDZ1 (PDB ID: 1G9O). We searched PDB database with Ska program [49] to find a PDZ domain that is complexed with a peptide and displays a high structural similarity with each PDZ domain. Once the best match had been found for each PDZ domain, it was substituted by a structurally superimposed NHERF1-PDZ1. The peptide in the crystal structure was then mutated into the sequence for the NHERF1-PDZ1-binding peptide using Chimera [50] . The resulting PDZ–peptide complex was subjected to FlexPepDock, a refinement tool with high-resolution peptide docking protocol, implemented within the Rosetta framework [51] . For generation of the model of PDZ in complex with peptide and cholesterol, a cholesterol molecule was docked sequentially to the PDZ–peptide complex using the package DOCK 6. How to cite this article : Sheng R. et al. Cholesterol modulates cell signaling and protein networking by specifically interacting with PDZ domain-containing scaffold proteins. Nat. Commun . 3:1249 doi: 10.1038/ncomms2221 (2012).